Sub-10 nm rutile titanium dioxide nanoparticles for efficient visible-light-driven photocatalytic hydrogen production Titanium dioxide is a promising photocatalyst for water splitting, but it suffers from low visible light activity due to its wide band gap. Doping can narrow the band gap of titanium dioxide; however, new charge-carrier recombination centres may be introduced. Here we report the design of sub-10 nm rutile titanium dioxide nanoparticles, with an increased amount of surface/sub-surface defects to overcome the negative effects from bulk defects. Abundant defects can not only shift the top of the valence band of rutile titanium dioxide upwards for band-gap narrowing but also promote charge-carrier separation. The role of titanium(III) is to enhance, rather than initiate, the visible-light-driven water splitting. The sub-10 nm rutile nanoparticles exhibit the state-of-the-art activity among titanium dioxide-based semiconductors for visible-light-driven water splitting and the concept of ultra-small nanoparticles with abundant defects may be extended to the design of other robust semiconductor photocatalysts. Since the discovery of water photolysis on a TiO 2 photoanode in the 1970s [1] , semiconductor photocatalysis has attracted significant attention due to its promising applications in environment remediation and solar energy conversion in the past decades [2] , [3] , [4] , [5] . TiO 2 is the initial semiconductor photocatalyst investigated and it is still regarded as a benchmark photocatalyst under ultravoilet irradiation due to its intrinsic high activity. However, TiO 2 is a type of wide band-gap semiconductor and it only adsorbs ultravoilet light, which greatly limits its practical applications [6] . Accordingly, persistent efforts have been made to narrow the band gap of TiO 2 to extend its working spectrum to the visible light region, that is, so-called band-gap engineering. Doping with metal or non-metal elements is known as a feasible means to tune the electronic structure of TiO 2 and to introduce new states into the TiO 2 band gap for visible light response [7] , [8] , [9] , [10] , [11] , [12] , [13] , [14] , [15] , [16] , [17] . In general, doping with non-metal elements, for example, C, N and S, can build acceptor states above the valence band from the p states of non-metal ions [16] , and doping with metal elements, for example, Fe and Cr, can build donor states below the conduction band [2] . For doped TiO 2 , the lattice defects induced by the dopants will unavoidably introduce new charge-carrier trapping and recombination centres, which might correspondingly show a degrading effect on the photocatalytic activity [7] . Moreover, doped TiO 2 materials are usually not adequate catalysts for photocatalytic hydrogen production from water splitting, although their superior activity in photocatalytic oxidation reactions have been well documented [6] , [18] . Self-doping with Ti 3+ was further developed for narrowing the band of TiO 2 without the introduction of unwanted carrier recombination centres from dopants [19] , [20] , [21] , which consequently exhibited good stability and considerable activity for photocatalytic hydrogen production under visible light [20] , [21] . Recently, hydrogenation of crystalline TiO 2 was disclosed as a new approach to enhance the visible as well as infrared light absorption of pristine TiO 2 and subsequently triggered great interest [22] , [23] , [24] , [25] , [26] , [27] , [28] . The surface disorder of hydrogenated black TiO 2 , instead of bulk Ti 3+ , was proposed to be responsible for the extended light absorption [23] , [24] . The hydrogenated TiO 2 exhibited remarkable activity in the photocatalytic hydrogen production from water splitting under full solar irradiation. However, considering that a sharp decline in the hydrogen production rate by two orders of magnitude (for example, from 10 to 0.1 mmol h −1 g −1 ) [22] , [25] was observed if ultraviolet light was filtered out ( λ >400 nm), the original hydrogen production activity should more probably come from the enhanced charge separation and transportation under ultraviolet irradiation rather than the extended visible light absorption [29] . The possibility of extending the working spectrum of TiO 2 to the visible light region is generally acknowledged based on both experimental observations and theoretical calculations [7] , [8] , [9] , [10] , [11] , [12] , [13] , [14] , [15] , [16] , [17] , [18] , [19] , [20] , [21] , [22] , [23] , [24] , [25] , [26] , [27] , [28] , [29] , [30] , [31] , [32] . The common point of different strategies lies in disrupting the integrity of ordered lattice structure of pristine TiO 2 (rutile or anatase) and building new states within the band gap for photoexcitation with lower energy. However, despite recent achievements, a simple strategy to TiO 2 -based semiconductors for efficient visible-light-driven photocatalytic hydrogen production is still challenging. Indeed, the successful photocatalyst system should fulfill all the requirements simultaneously: (i) narrowed band gap for visible light response; (ii) delicately designed band edge positions to realize photocatalytic redox reaction; and (iii) high efficiency for charge-carrier separation to promote photocatalytic activity. Here we present a direct hydrolysis route to sub-10 nm rutile TiO 2 nanoparticles for efficient photocatalytic hydrogen production under visible light irradiation. The simple strategy leads to state-of-the-art photocatalytic activity among TiO 2 -based semiconductors, and the simplified rutile TiO 2 semiconductor system can provide information on the essence of defect-induced visible light photocatalytic activity. Preparation and characterization of rutile TiO 2 samples Anatase and rutile TiO 2 , both with tetragonal structure, are commonly used in photocatalytic reactions. Rutile TiO 2 has a band gap ca. 0.2 eV lower than that of anatase (3.0 versus 3.2 eV), and this could be crucial to the band-gap narrowing to extend its working spectrum to the visible light region. Bulk rutile TiO 2 can be obtained via the high temperature calcination of anatase TiO 2 at temperatures higher than 773 K, while rutile TiO 2 nanostructures can be prepared via a hydrothermal route [33] , [34] or a direct hydrolysis route [35] , [36] , [37] . In the present work, the direct hydrolysis of TiCl 4 , free of any additives, is employed to prepare rutile TiO 2 nanoparticles. Experimentally, the hydrolysis of TiCl 4 solution (TiCl 4 /H 2 O=1:3 v/v) can produce rutile TiO 2 nanoparticles below 10 nm. We need to emphasize that the rapid hydrolysis and evaporation not only ensure the formation of rutile TiO 2 nanoparticles instead of nanorods in the presence of concentrated chloride ions but also create abundant defects in the as-obtained rutile TiO 2 nanoparticles (vide infra). As shown in Fig. 1a , the sample prepared via hydrolysis route followed by calcination at 473 K, T-1, and the reference sample prepared via hydrothermal route followed by calcination at 473 K, T-3, give the typical diffraction patterns of rutile TiO 2 (JCPDF#21-1276), indicating that pure rutile phase is obtained. The crystallinity of T-1 is relatively low and the crystallite size is calculated to be ca. 9 nm according to the Scherrer equation from the broadening of rutile (110) reflection. 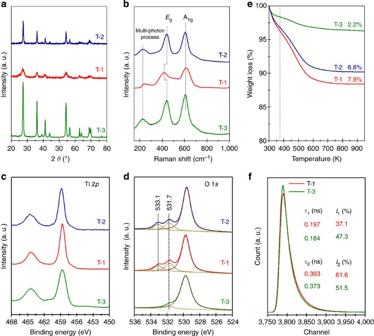Figure 1: Spectroscopy charatcerization of rutile TiO2samples. (a) XRD patterns of rutile TiO2samples. (b) Raman spectra of rutile TiO2samples. (c,d) Ti 2pand O 1sXPS of rutile TiO2samples. (e) Thermogravimetry analysis of rutile TiO2samples. (f) Positron annihilation lifetime spectra of rutile TiO2samples with corresponding positron lifetime and relative intensity in the inset. Calcination at 673 K can, on the one hand, greatly enhance the crystallinity of rutile TiO 2 but result in a significant increase in the crystallite size of T-2 ( Table 1 ). Raman spectra of the samples with relative high crystallinity, that is, T-2 and T-3, show three Raman-active modes of multi-proton process (230 cm −1 ), E g (440 cm −1 ) and A 1g (610 cm −1 ), corresponding to the tetragonal space group of P42/mnm [38] . For T-1, an obvious blue shift and broadening of the E g band (~25 cm −1 , Fig. 1b ) is clearly observed due to the photon-confinement effects induced by defects [23] , [39] . Figure 1: Spectroscopy charatcerization of rutile TiO 2 samples. ( a ) XRD patterns of rutile TiO 2 samples. ( b ) Raman spectra of rutile TiO 2 samples. ( c , d ) Ti 2 p and O 1 s XPS of rutile TiO 2 samples. ( e ) Thermogravimetry analysis of rutile TiO 2 samples. ( f ) Positron annihilation lifetime spectra of rutile TiO 2 samples with corresponding positron lifetime and relative intensity in the inset. Full size image Table 1 Physico-chemical properties of TiO 2 samples under study. Full size table X-ray photoelectron spectroscopy (XPS) analysis is performed to study the surface and sub-surface chemical states (in the depth up to 3 nm) of rutile TiO 2 samples. In Ti 2 p spectra ( Fig. 1c ), two peaks at binding energy of 458.6 and 464.1 eV, assignable to 2 p 3/2 and 2 p 1/2 , respectively, of Ti 4+ in TiO 2 (ref. 40 ), are observed for all rutile TiO 2 samples, indicating the identical chemical state of Ti atoms in these samples. No obvious Ti 3+ signals could be observed in Ti 2 p spectra. In O 1-s spectra ( Fig. 1d ), a well-formed peak at 529.6 eV and two shoulders at 531.7 and 533.1 eV are observed for samples prepared by hydrolysis. The binding energy value of 529.6 eV is attributed to the lattice oxygen in TiO 2 (ref. 23 ), while the binding energy values of 531.7 and 533.1 eV are attributed to bridging hydroxyls and physisorbed water, respectively [41] , [42] . Hydrothermal synthesized sample T-3 exhibits a week peak shape at 531.7 eV corresponding to bridging hydroxyl groups, revealing its fine crystal structure with few surface defects. The presence of bridging surface hydroxyls in rutile TiO 2 samples is further supported by Fourier transform infrared spectroscopy (FTIR) with the observation of strong broad band located at 3,425 cm −1 ( Supplementary Fig. 1 ). It is interesting to note that the percentages of hydroxyls in total oxygen species for T-1 is slightly higher than that of T-2, both much higher than that of hydrothermal-synthesized T-3 ( Table 1 ). This is further confirmed by the thermogravimetry analysis in Fig. 1e , where weight losses of 7.9% and 2.2% in the temperature range of 373–973 K are observed for T-1 and T-3, respectively. Positron annihilation is a well-established technique to study the defects in semiconductor materials and the lifetime of the positron is able to give information on the nature of various defects down to the p.p.m. level [43] . We have employed this technique to investigate the defects in rutile TiO 2 samples prepared via direct hydrolysis and hydrothermal synthesis, and the results are shown in Fig. 1f . Two different fitted curves are clearly observed and the corresponding fitting parameters, lifetime, τ 1 , τ 2 and τ 3 , with relative intensity, I 1 , I 2 and I 3 , are summarized in the inset. The longest lifetime component τ 3 is attributed to the annihilation of orthopositronium atoms formed in very large voids presented in the material [44] . The lifetime components τ 1 and τ 2 have been demonstrated to indicate the existence of point defects in the bulk phase and the defects located on the surface of the samples, respectively [45] , [46] . The lifetime τ 1 and τ 2 of T-1 is comparable with that of T-3, which indicates the similar nature of surface and bulk defects in both samples, as the nature of defects can influence the local electron density and subsequently influence the positron lifetime [47] . The value of I 2 / I 1 , reflecting the intensity ratio of surface to bulk defects, is calculated to be 1.66 for T-1, obviously higher than the 1.09 of T-3, indicating the rich of surface defects in sub-10 nm rutile TiO 2 nanoparticles prepared via hydrolysis. The morphology and structure of rutile TiO 2 samples are analysed by transmission electron microscopy (TEM), as shown in Fig. 2a . T-1 appears as aggregates of nanoparticles with an average diameter of ca. 8 nm. Calcination at 673 K results in a distinct increase in the crystallite size of rutile TiO 2 from 8 to 27 nm, basically in agreement with X-ray diffraction results. The reference sample T-3 appears as nanorods with an average diameter of 16 nm and a length of 70 nm. For rutile TiO 2 , (110) facet is the most stable facet with lowest formation energy [48] and it is observed as the dominant facet for all rutile TiO 2 samples, as illustrated by the lattice fringes with a spacing of 0.325 nm in the high-resolution TEM images ( Fig. 2b ). In addition, disordered structure induced by defects, can be observed for rutile TiO 2 samples prepared via direct hydrolysis (T-3). Structural analysis based on high-resolution TEM image is further performed to provide visualized information on the existence of defects in rutile TiO 2 samples under study ( Fig. 2c ). For T-3, clearly resolved and well-defined lattice fringes are observed and the distance between the adjacent lattice planes is equivalent to standard spacing, revealing the high crystallinity and the formation of fine crystals. For T-1, different types of defects, including intrinsic bulk defects (different distances between adjacent lattice planes) and surface hydroxyls (higher intensity trace, as marked with circle in Fig. 2c ), can be clearly observed. Calcination at 673 K results in an increase in the crystallinity and the corresponding decrease in the defect degree. However, defects can still be observed, especially at the edges of nanoparticles ( Fig. 2c ), which is consistent with XPS results. Electron energy loss spectra (EELS) is further performed on T-1 and T-3, to give a qualitative interpretation of electronic states, as shown in Fig. 2d . For Ti L 2,3 edge, the Ti 3 d character splits into two groups: the threefold t 2g and the twofold e g orbitals, owing to the octahedral coordination with O atom forming s -type and π -type bonds [49] . The t 2g − e g splitting in Ti L 2,3 edge of T-1 and T-3 is quite similar, ruling out the existence of Ti with different electronic states, that is, Ti 3+ [23] . A noticeable intensity decrease of the L 2 peak of T-1 should be originated from the existence of defects [50] , [51] . 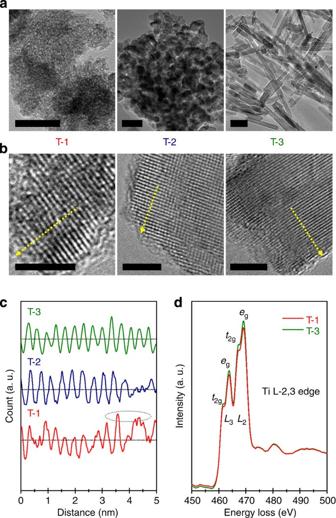Figure 2: Morphology and structure of rutile TiO2samples. (a) Overview TEM images of rutile TiO2samples. Scale bar, 50 nm. (b) High-resolution TEM (HRTEM) images of rutile TiO2samples. Scale bar, 4 nm. (c) Structural analysis based on HRTEM images, analysis region and orientation marked in the HRTEM images. (d) TiL2,3edge EELS of rutile TiO2samples. Figure 2: Morphology and structure of rutile TiO 2 samples. ( a ) Overview TEM images of rutile TiO 2 samples. Scale bar, 50 nm. ( b ) High-resolution TEM (HRTEM) images of rutile TiO 2 samples. Scale bar, 4 nm. ( c ) Structural analysis based on HRTEM images, analysis region and orientation marked in the HRTEM images. ( d ) Ti L 2,3 edge EELS of rutile TiO 2 samples. Full size image Band gap states of as-prepared rutile TiO 2 samples The optical properties of as-prepared rutile TiO 2 samples are investigated by diffuse reflectance ultraviolet–visible spectroscopy and the results are shown in Fig. 3a . T-3 shows a band-edge absorption around 410 nm, typical for rutile TiO 2 with a band-gap energy of ca. 3.0 eV. In contrast, T-1 shows obvious visible light absorption up to 600 nm, which should be originated from the existence of abundant defects. Calcination at 673 K will eliminate some of the defects (as discussed in the previous section) and therefore significantly reduce the absorption in visible light region. The plots of transformed Kubelka–Munk function versus the energy of light ( Fig. 3b ) give band-gap energies of 2.74, 2.84 and 2.98 eV for T-1, T-2 and T-3, respectively. Based on its light-absorption feature, the sub-10 nm rutile TiO 2 nanoparticles, T-1, should be an active photocatalyst under visible light irradiation. 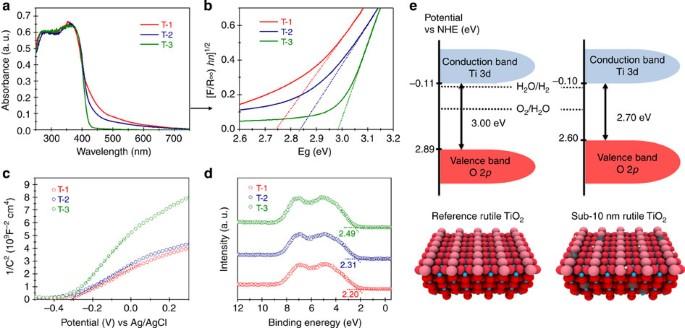Figure 3: Band-gap states of rutile TiO2samples. (a,b) Diffuse reflectance ultraviolet–visible spectra of rutile TiO2samples. (c) Mott–Schottky plots of rutile TiO2samples. (d) VB XPS of rutile TiO2samples. (e) Band energy diagram of reference (T-3) and sub-10 nm (T-1) rutile TiO2. Figure 3: Band-gap states of rutile TiO 2 samples. ( a , b ) Diffuse reflectance ultraviolet–visible spectra of rutile TiO 2 samples. ( c ) Mott–Schottky plots of rutile TiO 2 samples. ( d ) VB XPS of rutile TiO 2 samples. ( e ) Band energy diagram of reference (T-3) and sub-10 nm (T-1) rutile TiO 2 . Full size image To further address the relative band structure of rutile TiO 2 samples under study, the flat-band potential is measured using the electrochemical method in 0.5 M NaSO 4 solution (pH 6.8) and the Mott–Schottky plots are shown in Fig. 3c . The Mott–Schottky plots of all the rutile TiO 2 samples show a positive slope, which is typical for n -type semiconductors. The conduction band bottom of all rutile TiO 2 samples under study is quite similar ( ca . −0.10 eV versus normal hydrogen electrode) according to the Mott–Schottky plots. Moreover, T-1 shows a relatively smaller slope than T-3, indicating a faster charge transfer and a higher donor density [29] , [52] . The carrier densities ( N d ) of the samples can be calculated from the slopes of Mott–Schottky plots according to equation (1): [29] where e 0 is the electron charge (1.6 × 10 −19 C), ε is the dielectric constant of rutile TiO 2 , ε 0 is the permittivity of vacuum (8.86 × 10 −12 F m −1 ) and V is the applied bias at the electrode. The carrier densities are calculated to be 1.10 × 10 18 , 0.95 × 10 18 and 0.45 × 10 18 cm −3 for T-1, T-2 and T-3, respectively. As the defect sites always act as the electron donors, a higher carrier density implies the existence of a larger amount of defects. The valence band positions of rutile TiO 2 samples are determined by linear extrapolation of the leading edges of valence band (VB) XPS spectra to the base lines. As shown in Fig. 3d , apparent valence band values of 2.20, 2.31 and 2.49 eV are observed for T-1, T-2 and T-3, respectively. The scatterings of data relative to the fittings are proved to be <0.05 eV by repeated experiments. After calibration with reference Fermi level, actual valence band values of 2.60, 2.71 and 2.89 eV versus normal hydrogen electrode can be obtained for T-1, T-2 and T-3, respectively. Compared with T-3, T-1 shows ca . 0.3 eV upward shift in the valence band top, which is the origin of its visible absorption. To further clarify the influence of defects on the band structure of rutile, hybrid density functional theory (DFT) calculations were done with (2 × 2) rutile (110) slab models. The shifts of valence band top are summarized in Supplementary Table 1 . The existence of surface defects, both bridging hydroxyls and bridging oxygen vacancy on rutile (110), indeed induces upward shift of valence band top. Moreover, higher hydroxyl coverage results in stronger shift, which agrees with the experimental observation that the valence band top of T-1, with more bridging hydroxyl, is higher in T-3. However, a qualitative comparison is not easy in this study due to the simplified model used in DFT, that is, (1) extended surface in calculation versus nanoparticle in experiment and (2) single-type defects in calculation versus coexisted multi-type defects in experiment. Based on the results from Mott–Schottky plots ( Fig. 3c ) and VB XPS analysis ( Fig. 3d ), the band gaps are calculated to be 2.70, 2.82 and 3.00 eV for T-1, T-2 and T-3, respectively. These values are in good accordance with the band-gap values directly measured by ultraviolet–visible spectroscopy ( Supplementary Table 2 ). The detailed band diagrams of reference and sub-10 nm rutile TiO 2 are depicted in Fig. 3e . Compared with reference T-3, sub-10 nm T-1 exhibits similar conduction band bottom but distinct higher valence band top. Therefore, a band-gap narrowing of ca . 0.3 eV could be achieved, which indicates that T-1 is a promising visible-light photoactive semiconductor. Moreover, the band-edge position reveals that the T-1 is suitable for photocatalytic hydrogen production, as its conduction band bottom is more negative than the reduction potential of H 2 O/H 2 and its valence band top is more positive than the oxidation potential of O 2 /H 2 O. Photocatalytic hydrogen production from water splitting The photocatalytic activity of rutile TiO 2 samples (with 1 wt.% Pt as co-catalyst, Supplementary Fig. 2 ) was measured using the amount of hydrogen production from water splitting under different irradiations, and the time course of hydrogen evolution is shown in Fig. 4 . Under ultraviolet light ( Fig. 4a ), T-1 exhibits the highest mass-specific activity (24.7 mmol h −1 g −1 ), followed by T-3 (15.4 mmol h −1 g −1 ) and then T-2 (9.2 mmol h −1 g −1 ). It is surprising to note that T-1 with more defects exhibits distinctly higher photocatalytic activity than T-2 with less defects, considering that defects are generally regarded as the charge-carrier trapping and recombination centres. Under visible light (400 nm< λ <780 nm, Fig. 4b ), T-1 exhibits the highest mass-specific activity (932 μmol h −1 g −1 ), followed by T-2 (372 μmol h −1 g −1 ) and then T-3 (117 μmol h −1 g −1 ), consistent with their ability to absorb the visible light. Indeed, the hydrogen evolution rate achieved on T-1 is much greater, that is, more than five times higher, than other TiO 2 -based photocatalysts ever reported. A direct comparison between TiO 2 -based materials for visible-light-driven hydrogen production is summarized in Supplementary Table 3 . Under the irradiation of full-spectrum simulator, that is, sunlight air mass T-1 also exhibits a remarkable photocatalytic activity with a hydrogen evolution rate of 1,954 μmol h −1 g −1 , 4.2 and 5.6 times higher than that of T-2 and T-3, respectively ( Fig. 4c ). This value is also more than three times higher than reference TiO 2 P25. For a more objective comparison between the photocatalytic efficiencies for hydrogen production under visible light, the apparent quantum yield (QY) was calculated. The highest QY of 3.52% is obtained on T-1 sample under monochromatic light at λ =405 nm, followed by 1.40% of T-2 and 0.36% of T-3, consistent with the trend in photocatalytic activity under visible light ( Fig. 4b ). Moreover, high QY of 1.74% can be obtained on T-1 sample under monochromatic light at λ =420 nm. To our knowledge, these are the highest QYs ever reported for stable oxide semiconductors under comparable conditions [18] , [53] , although they are still lower than other systems, for example, CdSe nanocrystals capped with dihydrolipoic acid [54] and Ni-decorated CdS nanorods [55] . 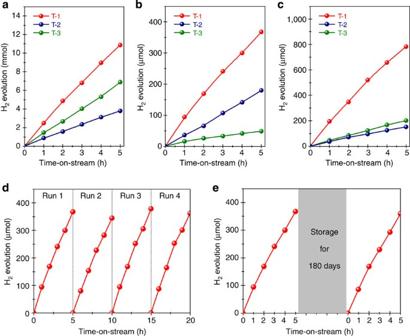Figure 4: Photocatalytic H2production over platinized rutile TiO2. (a) Under ultraviolet light, 320 nm<λ<400 nm. (b) Under visible light, 400 nm<λ<780 nm. (c) Under sunlight air mass 1.5 irradiation. (d) Cycling tests of T-1 under visible light. (e) Photcatalytic activity of T-1 after long-term storage, under visible light. Pt (1 wt%) isin situphoto-deposited on the surface of samples as the co-catalyst and 10 ml methanol is used as sacrificial reagent for water splitting. Figure 4: Photocatalytic H 2 production over platinized rutile TiO 2 . ( a ) Under ultraviolet light, 320 nm< λ <400 nm. ( b ) Under visible light, 400 nm< λ <780 nm. ( c ) Under sunlight air mass 1.5 irradiation. ( d ) Cycling tests of T-1 under visible light. ( e ) Photcatalytic activity of T-1 after long-term storage, under visible light. Pt (1 wt%) is in situ photo-deposited on the surface of samples as the co-catalyst and 10 ml methanol is used as sacrificial reagent for water splitting. Full size image In addition to its remarkable photocatalytic activity, T-1 exhibits very good stability as a photocatalyst. As shown in Fig. 4d , no noticeable decrease in the activity for photocatalytic hydrogen production can be observed in the cycling tests. Moreover, no obvious activity loss can be observed for T-1 even after conventional storage (sealed in glass sample bottle with finger tight) for as long as 180 days ( Fig. 4e ). Therefore, the remarkable activity and stability make T-1 a promising semiconductor photocatalyst for hydrogen production from water splitting under visible light or solar light. Functionalities of defects in rutile TiO 2 nanoparticles For sub-10 nm rutile nanoparticles T-1, the presence of abundant defects is clearly revealed by Raman, FTIR, XPS, photoluminescence and positron annihilation lifetime spectroscopy. The absence of reduced Ti states, for example, Ti 3+ , is confirmed by Ti 2 p XPS ( Fig. 1c ) and Ti L 2,3 -edge EELS ( Fig. 2d ). Therefore, the existence of oxygen vacancies or Ti interstitials, which are considered as major defects in TiO 2 contributing to band-gap states, could be expressly excluded. This is also supported by the fact that our rutile TiO 2 sample is exposed to ambient conditions with water and oxygen that would easily heal the oxygen vacancies and reduced Ti sites. Meanwhile, the presence of bridging hydroxyls is confirmed by O 1-s XPS ( Fig. 1d ) and FTIR analysis ( Supplementary Fig. 1 ). As the bridging hydroxyls are known to come from the dissociative adsorption of water on oxygen vacancies [56] , [57] , the detectable hydroxyls should indicate the ever-existing oxygen vacancies, together with Ti 3+ . That is, oxygen vacancies could be created during the synthesis of sub-10 nm rutile TiO 2 nanoparticles via fast hydrolysis, but they immediately react with water to form hydroxyls (O b −vac+O b +H 2 O→2OH b , where O b −vac means bridging oxygen vacancy, O b means bridging oxygen and OH b means bridging hydroxyl). In this context, hydroxyls should be the major defects in sub-10 nm rutile TiO 2 nanoparticles, also under ambient conditions, and the concentration of hydroxyls represents the defect degree in samples. The results from positron annihilation ( Fig. 1f ) and photoluminescence spectroscopy ( Supplementary Fig. 3 ) further indicate the presence of similar types of surface defects, that is, hydroxyls, of rutile TiO 2 prepared via both hydrolysis and hydrothermal routes. Thus, the only difference in rutile TiO 2 samples under study lies in their defect degrees, which directly influence the amount of upward shift in the valence band top ( Supplementary Table 1 ), and are responsible for the band-gap narrowing. The upward shift in the valence band top due to the existence of abundant defects in T-1 should be ascribed to the band bending [30] , most probably associated with charge imbalance induced by the defect energy levels [58] . Calcination at elevated temperature will eliminate some of the defects in T-1 and, therefore, reduce the extent of upward shift in the valence band top of T-2 ( Fig. 3d ). On the other hand, the defects in TiO 2 may greatly influence the efficiency of charge-carrier separation and the corresponding photocatalytic activity. The bulk defects will introduce charge-carrier trapping and recombination sites, and show degradation effects on the photocatalytic activity. In contrast, surface and sub-surface defects may contribute to charge-carrier separation, as the charges at surface or shallow traps become available for photocatalytic reaction. For most TiO 2 -based semiconductor materials reported, for example, doped TiO 2 , high defect degrees play a negative role on the photocatalytic activity, because the number of bulk defects is generally much higher than that of surface and sub-surface defects. As discussed above, more surface and sub-surface defects are desired for band-gap narrowing, while less bulk defects are wanted to promote the charge carrier separation. In general, the degrading effects from bulk defects will negate the increased visible light absorption from band-gap narrowing induced by surface defects and low visible-light-driven photocatalytic activity will be observed. In this study, we present a new concept to solve the problem by reducing the size of TiO 2 nanoparticles. With decreasing particle size, the ratio of surface to bulk increases, indicating the increased ratio of surface/sub-surface to bulk defects ( Fig. 1f ). Band-gap broadening due to quantum size effect, expressed as equation (2), could be neglected with TiO 2 particle size of >3 nm [59] , [60] . For T-1 with an average diameter of ca . 8 nm employed in this study ( Fig. 2a ), the positive effects from surface/sub-surface defects is strong enough to overcome the negative effects from bulk defects due to the relative high percentage of surface/sub-surface. This is well confirmed by its remarkable photocatalytic activity in hydrogen production under ultraviolet light ( Fig. 4a ). Taking the functionalities of defects on both band-gap narrowing and charge-carrier separation into consideration, we successfully develop the sub-10 nm rutile TiO 2 nanoparticles for efficient visible-light-driven photocatalytic hydrogen production. The visible light response of sub-10 nm rutile TiO 2 nanoparticles is first created via the introduction of abundant defects and then promoted by the specific defect distribution in nanoparticles and the use of co-catalyst Pt as well. If rutile TiO 2 with smaller particles size can be synthesized, higher visible-light-driven photocatalytic activity could be expected. Role of Ti 3+ in photocatalytic hydrogen production The role of Ti 3+ in the visible-light photocatalytic activity of TiO 2 -based materials has been intensively debated in the literature [17] , [20] , [21] , [22] , [23] , [24] , [61] . The major issue is that the appearance of Ti 3+ is always accompanied by defects and, therefore, will inevitably compound the problem. For our as-prepared rutile TiO 2 samples, the existence of lower oxidation states of Ti, that is, Ti 3+ , can be excluded based on XPS analysis. However, the presence of Ti 3+ can be clearly observed for all rutile samples on ultraviolet irradiation, as confirmed by the distinct electron spin resonance (ESR) signal at g 1 =1.972 and g 2 =1.949 ( Fig. 5a ) [20] , [62] . We then measured the quasi in situ ultraviolet–visible spectra of T-1 and T-3 for further information. As shown in Fig. 5b , the presence of Ti 3+ can be verified by the additional absorption in the visible light region for both T-1 and T-3 after 5 min time-on-stream ultraviolet irradiation to create a sufficiently detectable amount of Ti 3+ (ref. 63 ). Judging from the intensity of absorption intensity, we propose that more Ti 3+ species are presented in sub-10 nm rutile TiO 2 nanoparticles T-1 than reference T-3 on ultraviolet irradiation, which is clearly confirmed by the different intensities of Ti 3+ signals in ESR spectra ( Fig. 5a ). That is, the presence of defects in rutile TiO 2 should facilitate Ti 3+ formation during photocatalytic reaction under ultraviolet irradiation. 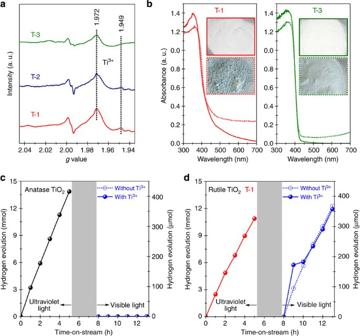Figure 5: Existence and role of Ti3+in photocatalytic hydrogen production. (a) ESR spectra of rutile TiO2samples under ultraviolet irradiation. (b) Quasiin situultraviolet–visible spectra of platinized rutile TiO2during photocatalytic hydrogen production from water splitting under ultraviolet irradiation; solid line: ultraviolet–visible spectrum before irradiation; dashed line: ultraviolet–visible spectrum after ultraviolet irradiation for 5 min; inset: photographs of samples before and after 5 min reaction). (c,d) Step responses of photocatalytic activity of platinized anatase and rutile TiO2to the change of irradiation light from ultraviolet light (400 nm>λ>320 nm) to visible light (780 nm>λ>400 nm). Figure 5: Existence and role of Ti 3+ in photocatalytic hydrogen production. ( a ) ESR spectra of rutile TiO 2 samples under ultraviolet irradiation. ( b ) Quasi in situ ultraviolet–visible spectra of platinized rutile TiO 2 during photocatalytic hydrogen production from water splitting under ultraviolet irradiation; solid line: ultraviolet–visible spectrum before irradiation; dashed line: ultraviolet–visible spectrum after ultraviolet irradiation for 5 min; inset: photographs of samples before and after 5 min reaction). ( c , d ) Step responses of photocatalytic activity of platinized anatase and rutile TiO 2 to the change of irradiation light from ultraviolet light (400 nm> λ >320 nm) to visible light (780 nm> λ >400 nm). Full size image To obtain a direct evidence on the role of Ti 3+ in the photocatalytic hydrogen production, step-response photocatalytic experiments are performed. Under ultraviolet light, anatase TiO 2 nanoparticles ( Supplementary Fig. 4 ) are highly active in photocatalytic water splitting with a hydrogen evolution rate of 31.2 mmol h −1 g −1 ( Fig. 5c ), slightly higher than the 24.7 mmol h −1 g −1 from sub-10 nm rutile TiO 2 nanoparticles ( Fig. 5d ). During photocatalytic reaction under ultraviolet irradiation, the presence of Ti 3+ is quite obvious with blue colouration (inset of Fig. 5b and Supplementary Fig. 5 ) [63] , [64] . After a 5-h photocatalytic reaction under ultraviolet radiation, the reaction system was either evacuated to preserve Ti 3+ or exposed to oxygen and then evacuated to eliminate Ti 3+ . In both cases, the anatase TiO 2 does not exhibit any detectable activity in subsequent photocatalytic hydrogen production tests under visible light ( Fig. 5c ). Therefore, it is rational to propose that the existence of Ti 3+ itself will not initiate the visible light photocatalytic activity for hydrogen production. This is consistent with the fact that the band-gap state created by Ti 3+ 3 d 1 state is about 1.0 eV below the conduction band of TiO 2 (ref. 32 ), which is obviously not suitable for H 2 O reduction to hydrogen ( Fig. 2e ). Sub-10 nm rutile TiO 2 , that is, T-1, is treated in the same manner and it exhibits remarkable photocatalytic activity under visible light after both treatments ( Fig. 5d ), which is ascribed to the surface defects, that is, hydroxyls, enabling the upward shift of valence band top of rutile TiO 2 . We also observe that T-1 with a significant Ti 3+ concentration exhibits much higher initial visible-light photocatalytic activity than that without Ti 3+ (time-on-stream of 1 h, hydrogen evolution rate from 967 to 1,763 μmol h −1 g −1 ). The photocatalytic activity becomes almost the same after a time-on-stream of 2 h. The presence of Ti 3+ can enhance the initial visible-light photocatalytic activity most probably due to the promoted methanol adsorption and/or the enhanced light absorbance and scattering [65] , and the promotional effects gradually fade away with the elimination of Ti 3+ . Consequently, we conclude that the presence of Ti 3+ cannot initiate visible-light photocatalytic activity in hydrogen production, but Ti 3+ is able to enhance the visible-light photocatalytic activity due to the promoted methanol adsorption. In summary, we have successfully developed a simple and scalable hydrolysis route to sub-10 nm rutile TiO 2 nanoparticles with diameters below 10 nm. We achieve a state-of-the-art hydrogen evolution rate of 932 μmol h −1 g −1 under visible light (>400 nm) and 1,954 μmol h −1 g −1 under simulated solar light with platinized sub-10 nm rutile TiO 2 nanoparticles (1 wt.% Pt) among TiO 2 -based semiconductors. Spectroscopic characterization results clearly confirm the existence of abundant surface defects, that is, hydroxyls, in the as-prepared rutile TiO 2 nanoparticles, which is responsible for the band-gap narrowing. The sub-10 nm particle size increases the percentage of surface/sub-surface defects compared with bulk defects, which results in enhanced charge-carrier separation. Moreover, we have revealed that the existence of defects in rutile TiO 2 is in favour of Ti 3+ formation during the photocatalytic reaction under ultraviolet irradiation. The presence of Ti 3+ cannot initiate the visible-light photocatalytic activity, but it is able to enhance the visible-light-driven water splitting most likely due to the promoted reagent adsorption. The results presented here provide new insights into the functionalities of defects in visible-light photocatalytic activity. The concept of ultra-small nanoparticles should be useful for the future design of robust semiconductor photocatalysts with tunable band gap. Preparation of rutile TiO 2 All of the chemical reagents of analytical grade were purchased from Alfa Aesar Chemical Co. and used as received without further purification. In a typical hydrolysis synthesis of rutile TiO 2 , 10 ml titanium tetrachloride (TiCl 4 ) was dropwise added into 30 ml ice water under stirring to prepare a transparent TiCl 4 aqueous solution. After further stirring for 30 min, the TiCl 4 aqueous solution was rapidly heated to 373 K (within 5 min) to remove the water and hydrogen chloride (Note: Rapid heating is crucial to obtain rutile TiO 2 nanoparticles). The obtained white solid was thoroughly washed with deionized water, followed by drying in air at 353 K for 24 h and calcination in a muffle furnace at temperatures of 473 or 673 K for 2 h. The final products are denoted as T-1 and T-2, respectively. For reference, rutile TiO 2 was also prepared via a hydrothermal route. Typically, 10 ml of 1 M TiCl 4 aqueous solution was added to 50 ml water and the resulting solution was directly transferred into a 75-ml Teflon-lined autoclave for static crystallization at 453 K for 24 h. The resulting precipitates after crystallization were separated from the liquid phase by centrifugation, thoroughly washed with water, dried at 353 K for 24 h, subjected to calcination at 473 K for 2 h and denoted as T-3. For the synthesis of anatase TiO 2 , TiCl 4 was dropwise added into ice water under stirring to prepare a TiCl 4 aqueous solution with concentration of 1 mol l −1 . Next, 30 ml of TiCl 4 aqueous solution was mixed with 30 ml of KOH solution (1 mol l −1 ) and the resulting solution was transferred into a 75-ml Teflon-lined autoclave for static crystallization at 373 K for 24 h. The resulting precipitates after crystallization were separated from the liquid phase by centrifugation, thoroughly washed with water, dried at 353 K for 24 h, subjected to calcination at 473 K for 2 h and denoted as T-4. Characterization techniques The specific surface areas of TiO 2 samples were determined through N 2 adsorption/desorption isotherms at 77 K collected on a Quantachrome iQ-MP gas adsorption analyser. The X-ray diffraction patterns of TiO 2 samples were recorded on a Bruker D8 ADVANCE powder diffractometer using Cu-Kα radiation ( λ =0.1542, nm) at a scanning rate of 4° per min in the region of 2 θ =20–80°. Raman analysis was carried out on a Renishaw InVia Raman spectrometer and the spectra were obtained with the green line of an Ar-ion laser (514.53 nm) in micro-Raman configuration. Diffuse reflectance ultraviolet–visible spectra of TiO 2 samples ( ca. 20 mg diluted in ca . 80 mg BaSO 4 ) were recorded in the air against BaSO 4 in the region of 200–700 nm on a Varian Cary 300 ultraviolet–visible spectrophotometer. For the so-called quasi in situ ultraviolet–visible spectroscopy, 50 mg platinized TiO 2 (1 wt.% Pt) was mixed with 10 ml methanol aqueous solution (10%) in a home-made quartz reaction chamber, evacuated and then sealed for analysis. The diffuse reflectance ultraviolet–visible spectra against BaSO 4 were recorded before and after ultraviolet light irradiation for 10 min on the Varian Cary 300 ultraviolet–visible spectrophotometer. The concentration of surface hydroxyls in rutile TiO 2 was analysed by thermogravimetry on a Setram Setsys 16/18 thermogravmetric analyser. In a typical measurement, 0.1 g of rutile TiO 2 sample was heated in an Al 2 O 3 crucible from 300 to 973 K with a constant heating rate of 10 K min −1 and under flowing Ar of 20 ml min −1 . TEM images were taken on a FEI Tecnai G2 F20 electron microscope at an acceleration voltage of 200 kV and a Tecnai G2 F30 electron microscope at an acceleration voltage of 300 kV. A few drops of alcohol suspension containing the sample were placed on a carbon-coated copper grid, followed by evaporation at ambient temperature. EELS spectra of samples were collected using a GIF Tridiem 863 analyser. The lattice structural analysis was done using the Digital Micrograph software. XPS spectra of samples were recorded on a Kratos Axis Ultra delay line detector spectrometer with a monochromated Al-Kα X-ray source (hν=1486.6 eV), hybrid (magnetic/electrostatic) optics and a multi-channel plate and delay line detector. All spectra were recorded using an aperture slot of 300 × 700 μm. Survey spectra were recorded with a pass energy of 160 eV and high-resolution spectra with a pass energy of 40 eV. Accurate binding energies (±0.1 eV) were determined with respect to the position of the adventitious C 1 s peak at 284.8 eV. VB XPS of samples were measured on PHI Quantera XPS Scanning Microprobe spectrometer using Al-Kα X-ray source (hν=1486.6 eV). The energy scales are aligned by using the Fermi level of the XPS instrument (4.10 eV versus absolute vacuum value). Mott–Schottky plots were obtained using a three-electrode cell electrochemical workstation (IVIUM CompactStat). The saturated Ag/AgCl and platinum foil (2 × 2 cm 2 ) were used as the reference electrode and the counter electrode, respectively. The sample of 1 mg TiO 2 was dispersed in 1 ml anhydrous ethanol and then evenly grinded to a slurry. The slurry was spread onto indium tin oxide glass and the exposed area was kept at 0.25 cm 2 . The prepared indium tin oxide/samples were dried overnight under ambient conditions and then used as the working electrode. The measurements were carried out at a fixed frequency of 1 kHz in 0.5 M Na 2 SO 4 solution in the dark. Positron annihilation experiments were performed on a fast–slow coincidence ORTEC system with a time resolution of 187 ps full width at half maximum. The sample powder was pressed into a disk (diameter: 10.0 mm, thickness: 1.0 mm). A 5 × 10 5 -Bq source of 22 Na was sandwiched between two identical sample disks. Measured spectra were analysed by the computer programme LT9.0, with source correction to evaluate the lifetime component τ i and corresponding intensity I i , using equation (3): ESR was carried out on a JEOL JES-FA200 cw-EPR spectrometer (X-band) with a microwave power of 1.0 mW and a modulation frequency of 100 kHz. Mn-Marker was used as an internal standard for the measurement of the magnetic field. In a typical experiment, sample of 150 mg was placed in a quartz ESR tube and evacuated at room temperature for 2 h. After cooling down to 110 K, the tube was analysed under ultraviolet irradiation. Photocatalytic hydrogen production from water splitting Photocatalytic water splitting with methanol as sacrificial agent was performed in a top-irradiation-type Pyrex reaction cell connected to a closed gas circulation and evacuation system under the irradiation of Xe lamp (PLS-SXE, wavelength: 300–2,500 nm) with different optical reflector or filter (UVREF: 320–400 nm, ca . 83 mW cm −2 ; UVCUT400: 400–780 nm, ca . 80 mW cm −2 ) or Air Mass 1.5 ( ca . 100 mW cm −2 ). In a typical experiment, catalyst sample of 100 mg was suspended in ca . 100 ml 10% methanol aqueous solution (10 ml methanol and 90 ml H 2 O) in the reaction cell. After being evacuated for 30 min, the reactor cell was irradiated by the Xe lamp at 200 W, at a constant temperature of 313 K under stirring. The gaseous products were analysed by an on-line gas chromatograph (Varian CP-3800) with a thermal conductivity detector. For all TiO 2 samples, 1 wt.% Pt was in situ photo-deposited from 1 M H 2 PtCl 6 aqueous solution as co-catalyst, resulting a pH value of 6.5 in the reaction system. The apparent QYwas measured using the same experimental setup for the photocatalytic hydrogen generation, but with additional band-pass filters to obtain monochromatic light at λ =405 nm or λ =420 nm (together with UVCUT400). The power density was measured to be ca . 2.0 ( λ =405 nm) or 1.5 mW cm −2 ( λ =420 nm) using a calibrated photodiode and the QY was calculated by equation (4): DFT calculations DFT calculations were performed with the plane-wave-based Vienna ab initio simulation package VASP [66] at hybrid level in form of HSE06 (ref. 67 ). The (2 × 2) rutile TiO 2 (100) was represented by periodic slab models of four tri-TiO 2 layer thick. The valence wave functions were expanded in a plane-wave basis with a cutoff energy of 400 eV, while the interaction between the atomic cores and the electrons was described by the projector augmented wave method [68] . A Monkhorst–Pack mesh [69] of 2 × 1 × 1 was used to sample the Brillouin zone during the geometry optimization (to 5 × 10 −4 eV pm −1 ), while the mesh was increased to 4 × 2 × 1 in density of state analysis. The bands of different defect slabs were aligned to the same vacuum level. How to cite this article : Li, L. et al . Sub-10 nm rutile titanium dioxide nanoparticles for efficient visible-light-driven photocatalytic hydrogen production. Nat. Commun. 6:5881 doi: 10.1038/ncomms6881 (2015).